Regulation of protein glycosylation and sorting by the Golgi matrix proteins GRASP55/65 The Golgi receives the entire output of newly synthesized cargo from the endoplasmic reticulum, processes it in the stack largely through modification of bound oligosaccharides, and sorts it in the trans -Golgi network. GRASP65 and GRASP55, two proteins localized to the Golgi stack and early secretory pathway, mediate processes including Golgi stacking, Golgi ribbon linking and unconventional secretion. Previously, we have shown that GRASP depletion in cells disrupts Golgi stack formation. Here we report that knockdown of the GRASP proteins, alone or combined, accelerates protein trafficking through the Golgi membranes but also has striking negative effects on protein glycosylation and sorting. These effects are not caused by Golgi ribbon unlinking, unconventional secretion or endoplasmic reticulum stress. We propose that GRASP55/65 are negative regulators of exocytic transport and that this slowdown helps to ensure more complete protein glycosylation in the Golgi stack and proper sorting at the trans -Golgi network. The Golgi apparatus has a central role in the trafficking and processing of membrane and secretory proteins in the exocytic and endocytic pathways, as well as in multiple recycling routes. It is present in almost all eukaryotic cells and is composed of stacks of flattened cisternae that are laterally linked to form a perinuclear ribbon-like structure in mammalian cells [1] . The Golgi matrix proteins, a group of proteins localized at the cytoplasmic face of the Golgi membranes, have important roles in Golgi stack and ribbon formation, membrane tethering, unconventional secretion, Golgi biogenesis during cell division, as well as cell cycle progression, apoptosis and directed cell migration [2] , [3] , [4] , [5] , [6] , [7] , [8] , [9] . Among these Golgi matrix proteins, two homologues, GRASP65 ( G olgi r e a ssembly s tacking p rotein of 65 kDa) and GRASP55 (55 kDa) were first discovered as Golgi stacking factors [10] , [11] . Antibodies against GRASP65 or GRASP55 inhibited postmitotic stacking of newly formed cisternae both in vitro [10] , [11] and in vivo [12] . Depletion of GRASP65 or GRASP55 in mammalian cells by RNA interference (RNAi) reduced the number of cisternae per stack [13] , [14] , [15] , and simultaneous depletion of both GRASPs resulted in complete disassembly of the Golgi stacks [14] . In Drosophila S2 cells, depletion of the sole Drosophila GRASP protein and its interacting protein, dGM130, resulted in the disassembly of the Golgi stacks into single cisternae and vesicles [16] . In addition to Golgi stacking, GRASP65 and GRASP55 have been shown to have other functions, including ribbon linking, cargo transport, unconventional secretion, cell cycle progression, apoptosis and Golgi remodelling in migrating cells [12] , [13] , [17] , [18] , [19] , [20] , [21] . GRASP65 and GRASP55 form homodimers and dimers from adjacent membranes further form trans -oligomers that tether membranes into close proximity [12] , [22] . GRASPs are localized between the cisternae, where their oligomers hold cisternal membranes into stacks [11] , [14] , [15] . It was also proposed that GRASPs localize to the rims of the Golgi stacks and link Golgi stacks into a ribbon [17] , [20] . GRASP65 may also exert its tethering function through its interacting protein GM130. This interaction is thought to participate in the docking of p115 tethered COPII vesicles [23] . It has also been shown that the GM130/GRASP65 complex recycles between the cis -Golgi and the late endoplasmic reticulum (ER)-Golgi intermediate compartment (ERGIC), the membrane station that dynamically protrudes from the Golgi and undergoes homotypic fusion with intermediate compartments [24] . Although the GRASP proteins have essential roles in Golgi structure formation, how they regulate Golgi functions has not been well studied. In our previous study, we inhibited the function of GRASP65 by microinjecting anti-GRASP65 antibodies into cells and we observed an increased rate of protein transport, probably due to the acceleration of vesicle formation from unstacked cisternae [25] . However, the microinjection technique used in this previous study did not allow us to perform the necessary biochemical and cell biology experiments to examine protein glycosylation, sorting and other cellular activities. In the present study, we knocked down GRASP55, GRASP65 or both proteins by RNAi and determined the changes in protein trafficking, glycosylation, and sorting. Our results reveal essential roles for GRASP55/65 in protein glycosylation and sorting. GRASP depletion does not cause apoptosis or ER stress To determine the biological roles of GRASP55/65, we knocked down GRASP55, GRASP65 or both proteins in rtTA HeLa m2 cells with RNAi as previously described [14] , [15] . The depletion was efficient, determined by immunofluorescence microscopy and western blot ( Supplementary Fig. S1 ). GRASP depletion had no significant effect on the cellular levels of coat proteins, Rabs and tethers, SNAREs, membrane fusion proteins, Golgi enzymes and other Golgi structural proteins in the cell except GM130, which is reduced when both GRASP55 and GRASP65 were depleted, consistent with a previous observation [14] . To determine if GRASP depletion causes apoptosis in our system as previously reported [13] , we stained non-permeabilized cells with annexin V-GFP (green fluorescent protein), a widely used marker for early apoptosis [26] , [27] . Cells treated with GRASP RNAi were not stained with annexin V, while cells treated with staurosporine, a known apoptosis inducer, were readily stained ( Fig. 1a ). Furthermore, neither nuclear fragmentation nor cleaved caspase 3 was detected in the GRASP-depleted cells ( Fig. 1a ). These results demonstrate that GRASP depletion does not cause apoptosis in the cells in the present study. 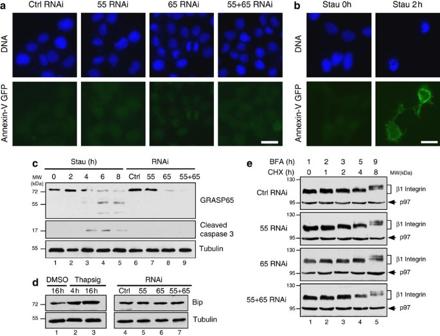Figure 1: Depletion of GRASP55/65 does not cause apoptosis or ER stress. (a) HeLa cells transfected with the indicated RNAi were stained with annexin V-GFP before fixation. Note that no obvious annexin V staining was observed on GRASP-depleted cells. (b) HeLa cells treated with 2 μM staurosporine (Stau) for 0 h or 2 h were stained with annexin V-GFP before fixation. Scale bars ina–b, 10 μm. (c) HeLa cells transfected with the indicated RNAi or treated with staurosporine (ST) were analysed by western blot. Note that the cleaved caspase 3 was detected after 2 h of staurosporine treatment, but not following the depletion of the GRASPs. (d) Depletion of GRASPs does not cause ER stress. HeLa cells transfected with the indicated RNAi or treated with dimethylsulphoxide or 2 μM thapsigargin (thapsig) for 4 h or 16 h were analysed by SDS–polyacrylamide gel electrophoresis and western blot. Note that the protein level of Bip increased after thapsig treatment, but not following GRASP depletion. (e) GRASP depletion does not result in ERAD. HeLa cells transfected with indicated RNAi were first treated with 5 μg ml−1Brefeldin A for 1 h followed by the addition of 100 μM cycloheximide (CHX) into the medium and incubated for the indicated time period. Shown are western blots of cell lysate for β1 integrin and p97 on the same gels. Molecular weight standards (kDa) are indicated on the left inc–e. Figure 1: Depletion of GRASP55/65 does not cause apoptosis or ER stress. ( a ) HeLa cells transfected with the indicated RNAi were stained with annexin V-GFP before fixation. Note that no obvious annexin V staining was observed on GRASP-depleted cells. ( b ) HeLa cells treated with 2 μM staurosporine (Stau) for 0 h or 2 h were stained with annexin V-GFP before fixation. Scale bars in a – b , 10 μm. ( c ) HeLa cells transfected with the indicated RNAi or treated with staurosporine (ST) were analysed by western blot. Note that the cleaved caspase 3 was detected after 2 h of staurosporine treatment, but not following the depletion of the GRASPs. ( d ) Depletion of GRASPs does not cause ER stress. HeLa cells transfected with the indicated RNAi or treated with dimethylsulphoxide or 2 μM thapsigargin (thapsig) for 4 h or 16 h were analysed by SDS–polyacrylamide gel electrophoresis and western blot. Note that the protein level of Bip increased after thapsig treatment, but not following GRASP depletion. ( e ) GRASP depletion does not result in ERAD. HeLa cells transfected with indicated RNAi were first treated with 5 μg ml −1 Brefeldin A for 1 h followed by the addition of 100 μM cycloheximide (CHX) into the medium and incubated for the indicated time period. Shown are western blots of cell lysate for β1 integrin and p97 on the same gels. Molecular weight standards (kDa) are indicated on the left in c – e . Full size image GRASP depletion also does not cause ER stress. Unlike thapsigargin-treated cells, Bip expression was not increased by GRASP depletion ( Fig. 1d ). We then determined whether GRASP depletion increases protein degradation in the ER. Cells were first treated with Brefeldin A to trap membrane and secretory proteins in the ER, and then treated with cycloheximide to block protein synthesis, and protein levels were measured by western blot. The reduction of β1 integrin, Lamp2 and cathepsin D over time in GRASP-depleted cells was comparable to control RNAi-treated cells ( Fig. 1e , Supplementary Fig. S2A,B ). In contrast, ER stress induced by thapsigargin treatment reduced the level of β1 integrin in the cell by ER-associated degradation (ERAD), an effect that was rescued by the proteasome inhibitor MG132 ( Supplementary Fig. S2C ). These results indicate that GRASP depletion does not cause ER stress or ERAD. GRASP depletion accelerates integrin trafficking To determine the roles of GRASP55/65 in protein trafficking, we performed pulse-chase experiments to examine the effects of GRASP depletion on the trafficking of α5 integrin, a type I transmembrane glycoprotein on the cell surface. Cells were labelled with 35 S-labelled methionine and cysteine followed by chases for different time periods. α5 integrin was then immunoprecipitated and analysed by autoradiography. After 0 h of chase, α5 integrin in all cells existed predominantly in their immature forms ( Fig. 2a ). After 2 h of chase, the mature form of α5 integrin, indicated by its higher molecular weight due to glycan processing in the Golgi, began to appear. Approximately 53% of the α5 integrin was detected as the mature form in the cells treated with control RNAi, while the proportion of the mature form increased to over 80% in cells depleted of GRASP55, GRASP65 or both. After 4 h and 6 h of chase, detectable amounts of immature α5 integrin existed in the control cells, whereas almost all of the α5 integrin had matured in the GRASP-depleted cells ( Fig. 2 ). These results demonstrate that GRASP depletion increases trafficking of plasma membrane proteins through the conventional trafficking route. 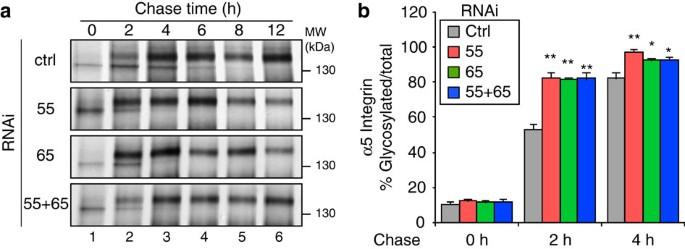Figure 2: Depletion of GRASPs accelerates α5 integrin trafficking. (a) GRASP depletion increases α5 integrin trafficking. HeLa cells transfected with the indicated RNAi were labelled with 250 μCi ml−1TRANS35S-LABEL for 1 h, chased for the indicated time periods, and lysed. α5 integrin were immunoprecipitated and analysed by SDS–polyacrylamide gel electrophoresis and autoradiography. Note that the mature form of α5 integrin appeared more rapidly in GRASP-depleted cells. (b) The ratio of the mature form versus total α5 integrin at the indicated chase time for one representative result out of three independent experiments. Shown are the quantitation results from three independent experiments.P-value was determined by Student’st-test; *P<0.05; **P<0.01; ***P<0.001 in this and all following figures. Note that the maturation rate of α5 integrin increased in GRASP-depleted cells. Figure 2: Depletion of GRASPs accelerates α5 integrin trafficking. ( a ) GRASP depletion increases α5 integrin trafficking. HeLa cells transfected with the indicated RNAi were labelled with 250 μCi ml −1 TRANS 35 S-LABEL for 1 h, chased for the indicated time periods, and lysed. α5 integrin were immunoprecipitated and analysed by SDS–polyacrylamide gel electrophoresis and autoradiography. Note that the mature form of α5 integrin appeared more rapidly in GRASP-depleted cells. ( b ) The ratio of the mature form versus total α5 integrin at the indicated chase time for one representative result out of three independent experiments. Shown are the quantitation results from three independent experiments. P -value was determined by Student’s t -test; * P< 0.05; ** P< 0.01; *** P <0.001 in this and all following figures. Note that the maturation rate of α5 integrin increased in GRASP-depleted cells. Full size image GRASP depletion accelerates VSV-G traffic through the Golgi To further dissect the effect of GRASP depletion on protein trafficking, we monitored the transport of the vesicular stomatitis virus glycoprotein (VSV-G) temperature-sensitive mutant (ts045) ( [28] ). Cells were infected with VSV-G ts045-GFP adenovirus at 40.5 °C for 16 h and then shifted to 32 °C to release VSV-G from the ER to the Golgi ( Supplementary Fig. S3 ). After 40.5 °C block, the VSV-G molecules in all cells were retained in the ER. After 15 min incubation at 32 °C, VSV-G started to accumulate in the Golgi and this process was accelerated in GRASP-depleted cells. After 30 min, the accumulation in GRASP-depleted cells was complete; whereas in control RNAi-treated cells, a significant amount of VSV-G was found in the ER. After 45 min, VSV-G containing vesicles emerged in GRASP-depleted cells but not in control RNAi-treated cells. After 60 min, VSV-G began to appear at the plasma membrane in GRASP-depleted cells, but not in control cells. These results demonstrate that GRASP depletion increases VSV-G trafficking through the Golgi. To quantitatively measure the traffic rate of VSV-G, we labelled VSV-G on the cell surface with an antibody against its extracellular domain and assessed the ratio of surface VSV-G to total VSV-G-GFP signal by flow cytometry 2 h after 32 °C release. As shown in Fig. 3a , the ratio of surface-to-total VSV-G was increased in the cells depleted of GRASP55, GRASP65 or both. These results are consistent with the previous observation that CD8 trafficking is accelerated in normal rat kidney (NRK) cells in which GRASP65 function is blocked by microinjected antibodies [25] . 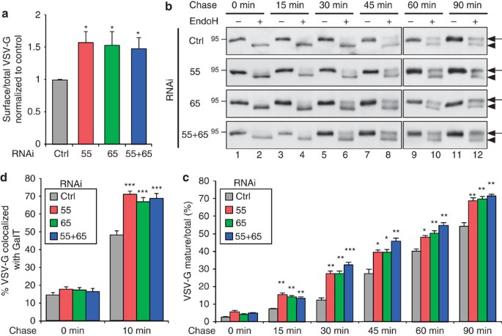Figure 3: GRASP depletion accelerates VSV-G trafficking through the Golgi membranes. (a) VSV-G traffic to the cell surface is accelerated by GRASP depletion. HeLa cells stably expressing VSV-G-ts045-GFP under an inducible promoter were transfected with control (ctrl), GRASP55 (55), GRASP65 (65), or both GRASP55 and GRASP65 (55+65) RNAi. The cells were incubated with doxycycline at 40.5 °C for 16 h to induce VSV-G expression and shifted to 32 °C for 120 min to release the VSV-G from the ER. The cells were collected, and the VSV-G on the surface was stained with an antibody against its extracellular domain followed by incubation with fluorescently labelled secondary antibodies. Total VSV-G and surface-bound VSV-G were assessed by flow cytometry. The ratio of surface-to-total VSV-G normalized against control cells (mean±s.e.m.) are shown based on three independent experiments. (b) GRASP depletion accelerates VSV-G trafficking. HeLa cells transfected with indicated RNAi were infected with VSV-G ts045-GFP adenovirus and incubated at 40.5 °C for 16 h. Cells were shifted to 32 °C, incubated for indicated time period (chase), and lysed. Proteins were treated with EndoH and analysed by western blot for VSV-G-GFP. Arrows indicate the EndoH resistant form and arrowheads indicate the EndoH sensitive form of VSV-G. Molecular weight markers are indicated on the left. (c) Quantitation of (b) to indicate the percentage of VSV-G in EndoH resistant form. Note that the difference between the GRASP-depleted cells and control RNAi-treated cells is most dramatic after 15–45 min chase when VSV-G travels through the Golgi membranes. (d) GRASP depletion accelerates VSV-G trafficking through the Golgi membranes. HeLa cells transfected with indicated RNAi were infected with VSV-G ts045-GFP adenovirus and incubated at 40.5 °C for 16 h. Cells were shifted to 15 °C for 2 h and then to 20 °C for 0 and 10 min followed by immunofluorescence microscopy. The co-localization of VSV-G with GalT was quantified with ImageJ. Shown are representative results (mean±s.e.m. from 20 different cells) from three independent experiments. Figure 3: GRASP depletion accelerates VSV-G trafficking through the Golgi membranes. ( a ) VSV-G traffic to the cell surface is accelerated by GRASP depletion. HeLa cells stably expressing VSV-G-ts045-GFP under an inducible promoter were transfected with control (ctrl), GRASP55 (55), GRASP65 (65), or both GRASP55 and GRASP65 (55+65) RNAi. The cells were incubated with doxycycline at 40.5 °C for 16 h to induce VSV-G expression and shifted to 32 °C for 120 min to release the VSV-G from the ER. The cells were collected, and the VSV-G on the surface was stained with an antibody against its extracellular domain followed by incubation with fluorescently labelled secondary antibodies. Total VSV-G and surface-bound VSV-G were assessed by flow cytometry. The ratio of surface-to-total VSV-G normalized against control cells (mean±s.e.m.) are shown based on three independent experiments. ( b ) GRASP depletion accelerates VSV-G trafficking. HeLa cells transfected with indicated RNAi were infected with VSV-G ts045-GFP adenovirus and incubated at 40.5 °C for 16 h. Cells were shifted to 32 °C, incubated for indicated time period (chase), and lysed. Proteins were treated with EndoH and analysed by western blot for VSV-G-GFP. Arrows indicate the EndoH resistant form and arrowheads indicate the EndoH sensitive form of VSV-G. Molecular weight markers are indicated on the left. ( c ) Quantitation of ( b ) to indicate the percentage of VSV-G in EndoH resistant form. Note that the difference between the GRASP-depleted cells and control RNAi-treated cells is most dramatic after 15–45 min chase when VSV-G travels through the Golgi membranes. ( d ) GRASP depletion accelerates VSV-G trafficking through the Golgi membranes. HeLa cells transfected with indicated RNAi were infected with VSV-G ts045-GFP adenovirus and incubated at 40.5 °C for 16 h. Cells were shifted to 15 °C for 2 h and then to 20 °C for 0 and 10 min followed by immunofluorescence microscopy. The co-localization of VSV-G with GalT was quantified with ImageJ. Shown are representative results (mean±s.e.m. from 20 different cells) from three independent experiments. Full size image To specifically analyse the effect of GRASP depletion on VSV-G trafficking through the Golgi membranes, we collected cell lysates at different points of 32 °C release and treated the samples with endoglycosidase H (endoH), an enzyme that removes mannose rich (ER/ cis -Golgi form) but not complex (Golgi and post Golgi form) N-linked oligosaccharides from glycoproteins. The change of a glycoprotein from endoH sensitive to endoH resistant has been widely used to monitor protein trafficking through the Golgi, while proteins transported by unconventional secretion bypass the Golgi and thus are not modified by Golgi enzymes [18] , [19] . Western blot showed that VSV-G trafficking is increased in GRASP-depleted cells compared with control cells ( Fig. 3b ). In control RNAi-treated cells, the endoH resistant form of VSV-G started to appear after 30 min chase and became stronger over time. In GRASP-depleted cells, the endoH resistant form of VSV-G appeared earlier (for example, after 15 min chase) and increased faster than that in control cells. The difference between GRASP-depleted cells and control cells was most obvious after 30 min and 45 min chase, the time period when VSV-G travelled through the Golgi stack ( Supplementary Fig. S3 ). To pinpoint the effect of GRASP depletion on VSV-G trafficking across the Golgi membranes, we first accumulated VSV-G in the ERGIC by incubating cells at 15 °C ( [29] ) and then shifted the cells to 20 °C to allow VSV-G to travel from the ERGIC to the trans Golgi [30] , [31] . Cells were analysed at different time points of 20 °C incubation by fluorescence microscopy for co-localization of VSV-G with galactosyltransferase-1 (GalT), a trans -Golgi marker. As shown in Fig. 3d , after 10 min incubation, 48.2±2.2% of VSV-G co-localized with GalT in control cells, while it was increased to 70.8±1.8%, 66.8±1.9% and 68.5±2.6% in cells depleted of GRASP55, GRASP65 or both GRASPs, respectively ( Fig. 3d ). Taken together, these results demonstrate that GRASP depletion increases protein trafficking through the Golgi membranes. GRASP depletion enhances coat protein membrane interaction To determine the mechanism of the enhanced protein trafficking by GRASP depletion, we assessed the effect of GRASP depletion on vesicle formation. By subcellular fraction ( Fig. 4a–f ), we found that membrane association of both β-COP and δ-COP, two subunits of the coatomer complex, significantly increased upon GRASP depletion. In addition to COPI, membrane association of clathrin heavy chain and the COPII component Sec31 also increased. These results are consistent with our previous data that unstacked Golgi membranes generate COPI vesicles more rapidly in an in vitro budding assay [25] . In addition, quantitation of electron microscope images of GRASP-depleted cells showed that GRASP depletion reduced the number of cisternae per stack [14] , [15] , but the average number of vesicles adjacent to each distinguishable Golgi stack in single-GRASP-depleted cells was significantly higher than in control RNAi-treated cells ( Fig. 4g ). Cells depleted of both GRASP55 and GRASP65 did not usually contain distinguishable Golgi stacks, with a large number of vesicles and single cisternae in the perinuclear region [14] . Collectively, these results demonstrate that GRASP depletion causes Golgi cisternal unstacking and enhances protein trafficking by stimulating vesicle formation. 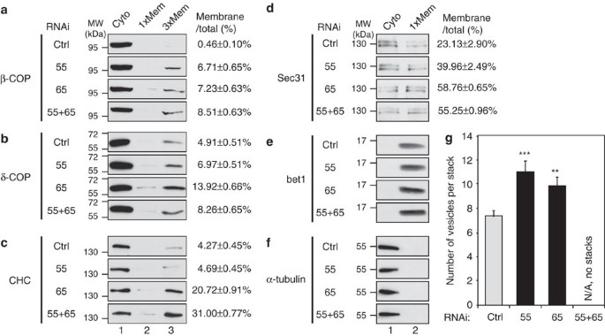Figure 4: GRASP depletion enhances membrane association of coat proteins. HeLa cells transfected with indicated RNAi were subjected to subcellular fractionation. Proteins in the cytosol and membrane fractions were analysed by western blot for β-COP (a), δ-COP (b), clathrin heavy chain (CHC,c), sec31 (d), bet1 (e) and α-tubulin (f). In some panels, three times of the membrane fractions were loaded onto the SDS–polyacrylamide gel electrophoresis (lane 3). Shown are representative images from three independent experiments. Quantification results (mean±s.e.m.) are shown on the right to indicate the percentage of the protein found in the membrane fractions. (g) GRASP depletion causes vesiculation of the Golgi. Quantitation of electron microscope images of GRASP-depleted cells for the number of vesicles adjacent to a Golgi stack. Shown are representative results (mean±s.e.m. from 20 different cells) from three independent experiments. Cells with both GRASP55 and GRASP65 depleted did not usually contain distinguishable Golgi stacks and thus were not quantified. Figure 4: GRASP depletion enhances membrane association of coat proteins. HeLa cells transfected with indicated RNAi were subjected to subcellular fractionation. Proteins in the cytosol and membrane fractions were analysed by western blot for β-COP ( a ), δ-COP ( b ), clathrin heavy chain (CHC, c ), sec31 ( d ), bet1 ( e ) and α-tubulin ( f ). In some panels, three times of the membrane fractions were loaded onto the SDS–polyacrylamide gel electrophoresis (lane 3). Shown are representative images from three independent experiments. Quantification results (mean±s.e.m.) are shown on the right to indicate the percentage of the protein found in the membrane fractions. ( g ) GRASP depletion causes vesiculation of the Golgi. Quantitation of electron microscope images of GRASP-depleted cells for the number of vesicles adjacent to a Golgi stack. Shown are representative results (mean±s.e.m. from 20 different cells) from three independent experiments. Cells with both GRASP55 and GRASP65 depleted did not usually contain distinguishable Golgi stacks and thus were not quantified. Full size image GRASP depletion impairs proper protein glycosylation As GRASP proteins slow the flow of cargo proteins, it was of interest to examine protein glycosylation in GRASP-depleted cells. To directly assess glycomic changes associated with GRASP depletion, we harvested N-linked glycans from control and GRASP-depleted cells, verified the structure of the most highly abundant high-mannose and complex glycans by multiple-stage mass spectrometry (MS n ), and quantified them relative to an external glycan standard ( Fig. 5a ). Depletion of both GRASP55 and GRASP65 resulted in a substantial decrease in N-linked glycoprotein glycans compared with that associated with equivalent amounts of proteins from control cells. Single-GRASP knockdowns showed somewhat variable increases or decreases in the abundance of individual glycans, although knockdown of GRASP55 was more consistently decreased in the major glycans. 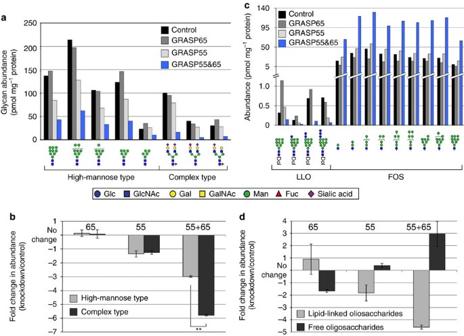Figure 5: Glycomic analysis of total protein glycosylation in GRASP-depleted cells. HeLa cells expressing RNAi targeting the indicated GRASP proteins were collected and processed for glycomic analysis by mass spectrometry. (a) The major high-mannose and complex glycans were quantified relative to an external standard and normalized to protein content. Double-knockdown cells exhibit significantly decreased glycan abundance. Glycan structural representations are consistent with the nomenclature proposed by the Consortium for Functional Glycomics: GlcNAc, blue square; Man, green circle; Gal, yellow circle; SA, purple diamond; Fuc, red triangle. (b) The fold change for each glycan indicated in panelawas calculated (knockdown/control). Average fold changes±s.e.m. are plotted; negative values indicate decreased abundance relative to control. Single knockdowns exhibit relatively minor alteration in the pool of major high-mannose and complex glycans, but the double-knockdown cells are significantly reduced in both high-mannose and complex glycans. In the double-knockdown cells, the fold-reduction in complex glycans is greater than the reduction in high-mannose glycans (Student’st-test, **P<0.001). (c) LLO and FOS were quantified by mass spectrometry relative to an external standard and normalized to protein content (Dol, dolichol pyrophosphate). Total LLO levels are significantly lower than FOS levels, note change inyaxis scale. All quantifiable LLO species were reduced in the GRASP double-knockdown cells, while some LLOs increased and some decreased relative to control in the single-knockdown cells. The abundance of all quantifiable FOS species was dramatically increased in double-knockdown cells, while single knockdown had relatively little effect on FOS levels. (d) Fold changes in LLO and FOS, calculated as inb, reveals the inverse relationship expected for precursor and product. Comparison with the fold change in glycoprotein glycan abundance (b) emphasizes that LLO availability limits glycosylation. When LLOs are decreased by knockdown, glycoprotein glycosylation is also decreased (55 alone and 55+65) and vice versa (65 alone), although the impact of either single knockdown is much smaller than the double knockdown. Figure 5: Glycomic analysis of total protein glycosylation in GRASP-depleted cells. HeLa cells expressing RNAi targeting the indicated GRASP proteins were collected and processed for glycomic analysis by mass spectrometry. ( a ) The major high-mannose and complex glycans were quantified relative to an external standard and normalized to protein content. Double-knockdown cells exhibit significantly decreased glycan abundance. Glycan structural representations are consistent with the nomenclature proposed by the Consortium for Functional Glycomics: GlcNAc, blue square; Man, green circle; Gal, yellow circle; SA, purple diamond; Fuc, red triangle. ( b ) The fold change for each glycan indicated in panel a was calculated (knockdown/control). Average fold changes±s.e.m. are plotted; negative values indicate decreased abundance relative to control. Single knockdowns exhibit relatively minor alteration in the pool of major high-mannose and complex glycans, but the double-knockdown cells are significantly reduced in both high-mannose and complex glycans. In the double-knockdown cells, the fold-reduction in complex glycans is greater than the reduction in high-mannose glycans (Student’s t -test, ** P< 0.001). ( c ) LLO and FOS were quantified by mass spectrometry relative to an external standard and normalized to protein content (Dol, dolichol pyrophosphate). Total LLO levels are significantly lower than FOS levels, note change in y axis scale. All quantifiable LLO species were reduced in the GRASP double-knockdown cells, while some LLOs increased and some decreased relative to control in the single-knockdown cells. The abundance of all quantifiable FOS species was dramatically increased in double-knockdown cells, while single knockdown had relatively little effect on FOS levels. ( d ) Fold changes in LLO and FOS, calculated as in b , reveals the inverse relationship expected for precursor and product. Comparison with the fold change in glycoprotein glycan abundance ( b ) emphasizes that LLO availability limits glycosylation. When LLOs are decreased by knockdown, glycoprotein glycosylation is also decreased (55 alone and 55+65) and vice versa (65 alone), although the impact of either single knockdown is much smaller than the double knockdown. Full size image To assess the efficacy of Golgi processing pathways in knockdown cell lines, the fold change in knockdown cells relative to control was calculated for each quantified high-mannose or complex glycan. By this parameter, the double knockdown exhibited a decrease in both high-mannose and complex glycans but the decrease in complex glycans was significantly greater than the decrease in high-mannose glycans (Student’s t -test, P <0.01, Fig. 5b ), consistent with the notion that GRASP depletion affects glycan processing in the Golgi. Fold changes for these glycan classes in single knockdowns did not reach statistical significance. Thus, GRASP depletion exerted two significant effects on glycoprotein processing: (1) decreased global N-linked glycoprotein glycosylation, and (2) decreased N-linked glycan complexity. Decreased N-glycosylation suggests altered co-translational initiation of glycoprotein glycosylation in the ER of GRASP-depleted cells. To determine whether decreased glycosylation resulted from reduced availability of N-linked oligosaccharide precursor or increased precursor hydrolysis, we measured the levels of dolichol-linked oligosaccharide (lipid-linked oligosaccharide, LLO) and free oligosaccharide (FOS) ( Fig. 5c ). Double-knockdown cells exhibited over fourfold decrease in LLO and threefold increase in FOS ( Fig. 5d ). Single-knockdown cells exhibited intermediate, less pronounced changes. These results indicate that GRASP proteins influence early secretory pathway function, a previously undetected activity of these proteins. GRASP depletion alters cell surface glycan presentation MS analysis of the total cellular glycome does not distinguish between intracellular and cell surface glycan presentation. To determine whether GRASP depletion affects the profile of glycans on the cell surface, we stained non-permeabilized cells with fluorescently labelled lectins. The Maackia amurensis (MAA) lectin binds to α(2,3) sialic acid (SA), a terminal capping monosaccharide residue on glycoproteins and glycosphingolipids [32] . The intensity of MAA staining decreased in cells depleted of GRASP55, GRASP65 or both, compared with control cells ( Fig. 6a versus 6b–d ). To verify this result, we mixed and cocultured control and GRASP55/65-depleted cells on the same coverslip and stained these cells for Wheat germ agglutinin (WGA), a lectin that selectively binds to SA and N-acetylglucosamine (GlcNAc). The cell surface signal for WGA was significantly reduced in GRASP-depleted cells compared with control cells ( Fig. 6e ). The effect of GRASP depletion on protein glycosylation was also confirmed by analysis of individual glycoproteins by SDS–polyacrylamide gel electrophoresis. We observed higher mobility of Lamp1 and Lamp2 on the gel upon GRASP depletion ( Fig. 6g ). Similar effects were observed by flow cytometry ( Supplementary Fig. S4A,B ) for cells surface-stained by MAA and the Sambucus nigra lectin that specifically binds to α(2,6) SA [32] . The staining pattern of Maclura pomifera , which binds to the O-linked core 1 disaccharide (Galβ1-3GalNAc or T-antigen), did not change significantly ( Supplementary Fig. S4C ), indicating that core 1 O-glycosylation is not significantly affected by GRASP depletion. These results demonstrate that GRASP depletion resulted in reduced protein glycosylation, but not reduced protein levels. 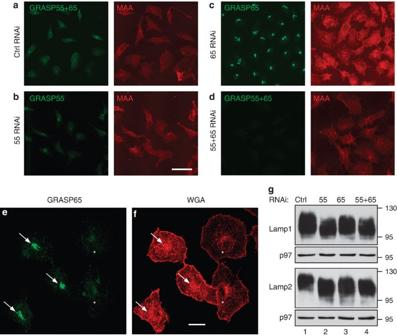Figure 6: Depletion of GRASP results in altered cell surface glycosylation. (a–d) Surface staining of fluorophore-conjugated lectin MAA specific for α(2,3) SA was reduced upon the depletion of GRASPs. Non-permeabilized HeLa cells treated with the indicated RNAi were exposed to tetramethylrhodamine isothiocyanate-conjugated MAA. The cells were then fixed, stained with GRASP antibodies and visualized using a confocal microscope. Scale bar, 50 μm. (e–f) HeLa cells transfected with control RNAi (arrows) and with RNAi for GRASP65 and 55 (asterisks) were mixed, cultured together and stained for GRASP65 (green) and WGA (red). Scale bar, 20 μm. (g) GRASP depletion impacts Lamp1 and Lamp2 glycosylation. Indicated GRASP-depleted cells were analysed for Lamp1, Lamp2 and p97 by western blots. Molecular weight markers are shown on the right. Note the shift of the bands after GRASP depletion. Figure 6: Depletion of GRASP results in altered cell surface glycosylation. ( a – d ) Surface staining of fluorophore-conjugated lectin MAA specific for α(2,3) SA was reduced upon the depletion of GRASPs. Non-permeabilized HeLa cells treated with the indicated RNAi were exposed to tetramethylrhodamine isothiocyanate-conjugated MAA. The cells were then fixed, stained with GRASP antibodies and visualized using a confocal microscope. Scale bar, 50 μm. ( e – f ) HeLa cells transfected with control RNAi (arrows) and with RNAi for GRASP65 and 55 (asterisks) were mixed, cultured together and stained for GRASP65 (green) and WGA (red). Scale bar, 20 μm. ( g ) GRASP depletion impacts Lamp1 and Lamp2 glycosylation. Indicated GRASP-depleted cells were analysed for Lamp1, Lamp2 and p97 by western blots. Molecular weight markers are shown on the right. Note the shift of the bands after GRASP depletion. Full size image GRASP depletion does not impact Golgi enzymes To determine whether the defects in glycoprotein glycosylation were caused by changes in glycan processing enzymes in the Golgi, we determined the expression level and localization of α-mannosidase II and GalT by western blot and microscopy. Our results showed that GRASP depletion did not affect the protein expression level and localizations of these Golgi enzymes ( Fig. 7 , Supplementary Figs S1,S5 ). 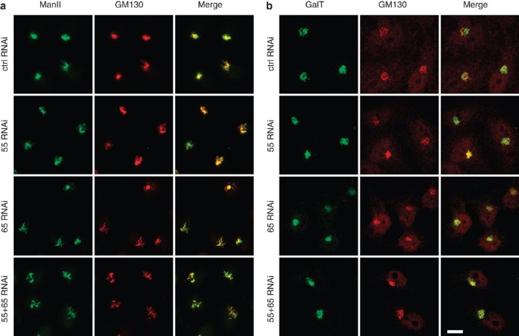Figure 7: GRASP depletion does not affect the localization of Golgi enzymes. HeLa cells were treated with the indicated RNAi and analysed by immunofluorescence microscopy for Mannosidase II (a), GalT (b) and GM130. Note that Golgi enzymes co-localized with GM130 in all cells. Scale bar, 10 μm. Figure 7: GRASP depletion does not affect the localization of Golgi enzymes. HeLa cells were treated with the indicated RNAi and analysed by immunofluorescence microscopy for Mannosidase II ( a ), GalT ( b ) and GM130. Note that Golgi enzymes co-localized with GM130 in all cells. Scale bar, 10 μm. Full size image GRASP depletion results in cathepsin D secretion We then determined the effect of GRASP depletion on protein sorting. Cathepsin D is synthesized in the ER as a 53-kDa polypeptide precursor; it is then transported through the Golgi to the lysosome, where the precursor is converted to a 47-kDa intermediate and, subsequently, the 31-kDa mature form [33] , [34] . Cathepsin D has previously been used as a marker for protein sorting [35] . Cells were incubated in serum-free media for 2 h, and cathepsin D in the cell lysate and media was detected by western blot. Three bands of cathepsin D were detected in the cell lysate, with the major band being the 31-kDa mature form; in contrast, only the 53-kDa immature form was detected in the media. Depletion of both GRASP55 and GRASP65 increased the amount of immature cathepsin D in the media by twofold ( Fig. 8a ). This was not due to cell lysis, as β-actin was not detected in the medium of these cells. These results suggest that disruption of the Golgi structure results in the missorting of cathepsin D to the extracellular space instead of the endosomes/lysosomes. In addition, the ratio between the intermediate and the immature form increased from 2 in control cells to 3–4 after GRASP depletion, indicating that the transport to the endosomes/lysosomes is enhanced when GRASP proteins are depleted ( Fig. 8a ). 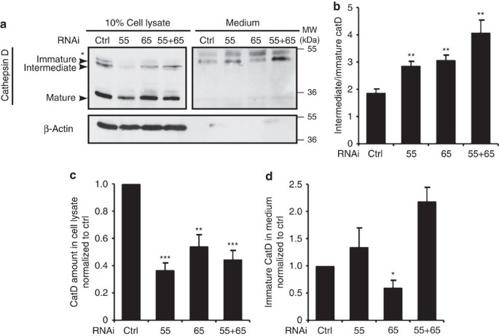Figure 8: GRASP depletion impairs cathepsin D sorting. (a) Missorting of cathepsin D in cells by GRASP depletion. HeLa cells transfected with the indicated RNAi were washed with PBS and incubated in serum-free DMEM for 2 h. The secreted proteins in the medium were trichloroacetic acid precipitated and normalized based on the total protein in the cell lysate. Equal portions of the cell lysate and medium were analysed by western blot for cathepsin D. Immature form: 53 kDa; intermediate form: 47 kDa; mature form: 31 kDa. The asterisk indicates a nonspecific band that appears in the medium. (b) Ratio of intermediate versus immature cathepsin D in cells transfected with the indicated RNAi by quantifying the related bands on the western blots ina. (c) The amount of cathepsin D in the cell lysate normalized to the cells transfected with control RNAi. (d) The amount of immature cathepsin D in the medium normalized to the cells transfected with control RNAi. The data are presented as the mean±s.e.m. of four independent experiments. Figure 8: GRASP depletion impairs cathepsin D sorting. ( a ) Missorting of cathepsin D in cells by GRASP depletion. HeLa cells transfected with the indicated RNAi were washed with PBS and incubated in serum-free DMEM for 2 h. The secreted proteins in the medium were trichloroacetic acid precipitated and normalized based on the total protein in the cell lysate. Equal portions of the cell lysate and medium were analysed by western blot for cathepsin D. Immature form: 53 kDa; intermediate form: 47 kDa; mature form: 31 kDa. The asterisk indicates a nonspecific band that appears in the medium. ( b ) Ratio of intermediate versus immature cathepsin D in cells transfected with the indicated RNAi by quantifying the related bands on the western blots in a . ( c ) The amount of cathepsin D in the cell lysate normalized to the cells transfected with control RNAi. ( d ) The amount of immature cathepsin D in the medium normalized to the cells transfected with control RNAi. The data are presented as the mean±s.e.m. of four independent experiments. Full size image The enhanced transport is not through Golgi ribbon unlinking GRASP65 and GRASP55 have been reported to have a role in Golgi ribbon formation [17] , [20] . Therefore, we determined whether Golgi ribbon unlinking was the cause for enhanced trafficking and reduced glycosylation by GRASP depletion. We induced Golgi ribbon unlinking by the depletion of golgin-84 (ref. 36 ) and by nocodazole treatment [37] , [38] , none of which induces Golgi unstacking. Both Golgin-84 depletion and nocodazole treatment caused significant Golgi ribbon unlinking and reduced VSV-G trafficking ( Supplementary Fig. S6 ), an opposite effect of GRASP depletion. Golgin-84 depletion also reduced glycosylation of Lamp1 and Lamp2, while Nocodazole treatment did not affect cell surface glycosylation. As depletion of GRASPs did not cause significant fragmentation of the Golgi or mislocalization of Golgi enzymes in our experimental system ( Fig. 7 ), these results rule out the possibility that the acceleration of protein trafficking by GRASP depletion is through Golgi ribbon unlinking. GRASP depletion does not induce unconventional secretion Previous studies indicate that GRASP65 and GRASP55 are involved in unconventional protein trafficking [18] , [39] , [40] . Under stress conditions, some proteins bypass the Golgi to the cell surface in a GRASP-dependent manner. Given that (1) GRASP depletion does not cause ER stress ( Fig. 1 , Supplementary Fig. S2 ), (2) GRASP depletion accelerates rather than slows down trafficking of the marker proteins ( Figs 2 , 3 ), (3) marker proteins used in this study (for example, integrins and VSV-G) travel through the Golgi and are glycosylated by Golgi enzymes ( Figs 2 , 3 , Supplementary Fig. S3 ), (4) membrane association of coat proteins involved in conventional traffic is enhanced in GRASP-depleted cells ( Fig. 4 ), and (5) GRASP depletion reduces the abundance of high-mannose glycans ( Fig. 5 ), unconventional secretion is unlikely to be the explanation of the observed effects. Finally, the role of GRASP65 and GRASP55 in unconventional secretion depends on their direct interaction with cargo proteins [18] . Therefore, we determined whether the marker proteins used in this study bind GRASP65 or GRASP55. As shown in Supplementary Fig. S7 , β1 integrin coimmunoprecipitated with α5 integrin, but not with GRASP55 or GRASP65. Similarly, Lamp1, Lamp2 and VSV-G did not interact with GRASP proteins, although GRASP65 coprecipitated with GM130. Taken together, these results demonstrate that the enhanced trafficking by GRASP deletion is not caused by unconventional secretion. Previous work has revealed multiple functions for GRASP55 and GRASP65 in Golgi structure formation and function, including Golgi cisternal stacking, ribbon linking, membrane tethering, protein trafficking, unconventional secretion and apoptosis [12] , [13] , [17] , [18] , [19] , [20] , [21] . However, a systematic determination of these functions in the same cellular context has not been reported. In this study, we depleted GRASP55, GRASP65 or both and explored the functional consequences. Depletion of GRASP proteins does not cause ER stress and apoptosis, but accelerates protein trafficking through the Golgi, decreases glycoprotein glycosylation and glycan complexity, and impairs protein sorting. GRASP depletion increases protein trafficking. We showed that the trafficking of VSV-G and α5 integrin was accelerated in GRASP-depleted cells using microscopy, EndoH digestion, flow cytometry and radioactive pulse-chase labelling. Notably, in the VSV-G experiment, the difference in VSV-G ts045-GFP transport between the control and GRASP RNAi-treated cells was most obvious at 30–45 min post temperature shift, the time when VSV-G travels through the Golgi. In contrast, surface VSV-G protein was more prominent 90–120 min after release in GRASP-depleted cells. The effect was significant though less obvious over the course of the longer chases, this may explain why previous studies did not detect the effect of GRASP65 or GRASP55 depletion on VSV-G transport [13] , [41] . Specifically, the EndoH treatment result pinpoints that VSV-G travels through the Golgi membranes faster in GRASP-depleted cells. Similarly, GRASP depletion also increased cathepsin D transport to the endosomal/lysosomal system. The enhanced protein trafficking by GRASP depletion is not caused by Golgi ribbon unlinking or unconventional secretion. Instead, it might be attributable, at least in part, to Golgi cisternal unstacking. Previously, we inhibited GRASP65 function by microinjection of GRASP65 antibodies into mitotic cells and monitored the transport of CD8 in postmitotic daughter cells. We showed that the Golgi become largely unstacked and CD8 arrived at the plasma membrane faster in cells with disassembled Golgi [25] . These observations were confirmed in GRASP-depleted cells in the present study. We hypothesize that when Golgi cisternae are fully stacked, vesicles can only form and fuse at the rims; once the cisternae begin to unstack, more membrane area becomes accessible, thereby increasing the rate of vesicle budding and cargo transport through the Golgi [25] . In support of this hypothesis, membrane association of coat proteins was increased in cells with unstacked Golgi membranes ( Fig. 4 ); unstacking also increased the rate of COPI vesicle formation from Golgi membranes in an in vitro budding assay [25] . On the other hand, vesicles that travel from one cisterna to the next in intact Golgi stacks may be held by tethering factors that reside on the surface of Golgi membranes, facilitating the fusion of vesicles with Golgi membranes. When the Golgi membranes become fully unstacked by the depletion of both GRASPs, the resulting membrane disorder may impair the function of these tethers. Thus, complete unstacking induced by double-GRASP knockdown may induce a significantly different organellar state than partial unstacking in the single-GRASP knockdown, perhaps explaining why we did not detect additive effects on protein trafficking when comparing the results of double- and single-GRASP depletion experiments. In general, our results do not contradict a role for GRASPs as Golgi stacking factors, but also indicate additional functions for these proteins [10] , [11] , [12] , [14] , [15] . GRASP depletion impairs proper protein glycosylation. By lectin binding and MS-based glycomic analysis, we found that GRASP depletion, especially the depletion of both GRASP65 and GRASP55, decreases glycoprotein glycosylation and glycan complexity ( Fig. 5b ). A reasonable explanation for the decrease in glycoprotein glycan complexity is that as cargo moves more rapidly through Golgi compartments, resident enzymes have less time to recognize and modify their substrates. As a result, glycoproteins contain more trimmed high-mannose glycans and less complex structures in the GRASP knockdown cells. Double knockdown has a more significant effect on glycan complexity than either single knockdown, despite the fact that trafficking rates are comparable in single and double knockdowns. Thus, glycan complexity must be affected by additional factors. For instance, Golgi organization is much more severely disturbed in double-knockdown cells, which may reflect impaired function of Golgi localized membrane tethers. As the expression and localization of a subset of Golgi enzymes are unaffected, it is more likely that altered glycosylation reflects changes in cargo trafficking, but not mislocalization or underexpression of Golgi enzymes. It is not immediately obvious why total N-linked glycan amount should be reduced in double-knockdown cells. Therefore, we examined the abundance and fate of LLO, the precursor donor substrates that present the Glc 3 Man 9 GlcNAc 2 glycan for en bloc transfer onto N-linked sequons of nascent glycoproteins. We detected decreased LLO abundance but increased FOS in GRASP double-knockdown cells ( Fig. 5 ). These results suggest that GRASP depletion increases LLO hydrolysis in the absence of ER stress or elevated ERAD. The role of GRASPs appears to be specific for N-glycosylation, as core 1 O-glycosylation in the ER is not significantly affected by GRASP depletion ( Supplementary Fig. S4C ). A role for GRASP in the early secretory pathway is consistent with our observation that upon GRASP depletion, the distribution of Sec31, a COPII coat, was also shifted towards the membrane-bound state ( Fig. 4 ), although its expression level was not affected ( Supplementary Fig. S1B ). In addition, the trafficking of VSV-G from the ER to the Golgi is enhanced upon GRASP depletion ( Supplementary Fig. S3 ). In Drosophila , Drosophila GRASP protein is localized to ER exit sites [16] ; in mammalian cells, GRASP65 is localized to the Golgi and ERGIC [24] , but has not been detected in the ER, which argues against a direct role for GRASPs in ER organization and function. Recent studies indicate novel influences of several protein kinases and small metabolic intermediates that, taken together, suggest the existence of novel regulatory mechanisms, which might underlie the pathophysiology of some congenital disorders of glycosylation in humans [42] , [43] , [44] , [45] , [46] . Therefore, we speculate that a feedback pathway monitors Golgi processing and adjusts the flux of protein trafficking and processing through early secretory compartments. Neither GRASP proteins nor Golgi stacking may be essential for protein trafficking and cell survival. The Golgi membranes in the budding yeast S. cerevisiae do not form stacks under normal growth conditions [47] . In yeast and other fungi, N-glycosylation in the Golgi mainly involves the addition of mannoses [48] , while in multi-cellular organisms N-glycosylation is more complex. Therefore, the multi-function of GRASP proteins and Golgi stacking may be features that were gained during evolution and have essential functions in multi-cellular organisms. Depletion of both GRASP55 and GRASP65 caused missorting of cathepsin D precursors to the extracellular space. This is possibly because of defective glycosylation, or due to the complete disruption of the Golgi stack and the sorting machinery in it. A similar observation has been reported in human mammary cancer cells upon oestrogen induction [49] . It is possible that stack formation ensures that sorting of cargo molecules occurs only when cargo molecules reach the trans -Golgi network (TGN), but not in other cisternae. Our results revealed that GRASP55/65 negatively regulate exocytic transport to ensure more complete glycosylation in the stack and better sorting at the TGN. In the Golgi stacks, GRASPs function as stacking factors. Depletion of the GRASP proteins results in Golgi cisternal unstacking [14] , [15] , increases membrane surface for vesicle formation, and accelerates protein trafficking [25] , but impairs protein glycosylation and sorting. Our results further suggest that Golgi cisternal stacking functions as a quality control mechanism for protein sorting and modifications by reducing the trafficking speed of cargo through the Golgi stack. Antibodies and reagents All reagents used were from Sigma, Roche or Calbiochem, unless otherwise stated. The following antibodies were used: monoclonal antibodies against Bet1, Gos28 and GM130 from BD Transduction Laboratories; monoclonal antibodies against β-actin (Sigma), clathrin heavy chain (Hong Chen), cleaved caspase 3 (Cell Signaling), ARF1 and β-COP (ref. 50 ), human β1,4 Galactosyltransferase I (CB002, CellMab AB), GFP antibody (Sigma), α5 integrin (BIIG2, DSHB), β1 integrin (P5D2, DSHB), Lamp1 (H4A3, DSHB), Lamp2 (H4B4, DSHB), α/β-SNAP and syntaxin 6 (ref. 51 ), α-tubulin (DSHB), and VSV-G extracellular domain (D. Sheff); polyclonal antibodies against Bip (P. Arvan), cathepsin D (sc-6486, Santa Cruz), human GRASP55 (Proteintech Group, Inc.), β1 integrin C-terminus (Abcam, EP1041Y), ManII (Kelley Moremen), Sec16 (X. Chen); polyclonal antibodies against δ- and ε-COP, GM130, and GRASP65, golgin-84, NSF, p47, p97, p115, Rab1, Sec31 and syntaxin 5 were previously described [51] , [52] . Lectin staining For immunofluorescence analysis, HeLa cells growing on cover slides were fixed in 3.7% paraformaldehyde. After blocking with 1% BSA (in PBS), surface glycosylated proteins were labelled with tetramethyl rhodamine isothiocyanate-conjugated lectins, such as MAA or WGA (EY laboratories), in the dark for 30 min at 4 °C. After washing with 1% BSA, the cells were permeabilized with 0.3% Triton X-100 and processed for immunofluorescence with the indicated antibodies. For flow cytometry analysis, HeLa cells were harvested in PBS containing 20 mM EDTA, blocked with cold BSA buffer, and labelled with FITC-conjugated lectins (EY laboratories) in the dark at 4 °C, for 30 min. After washing, the cells were fixed in 3.7% paraformaldehyde and analysed on a FACScalibur flow cytometer (BD Biosciences). Glycomic analysis HeLa cells transfected with control or GRASP RNAi were washed with cold PBS, scraped and collected by centrifugation. Proteins were harvested from the cell pellets as previously described [53] . Briefly, the cell pellets were resuspended in ice-cold water and disrupted by Dounce homogenisation on ice. The homogenate was adjusted to 4:8:3::chloroform:methanol:water before removal from ice. After 18 h of end-over-end agitation (Nutator), the insoluble proteinacious material was collected by centrifugation. Following re-extraction of the pellet three times with 4:8:3 and once with ice-cold 80% acetone (v/v, aqueous), the final pellet was dried under a gentle stream of nitrogen and stored as a fine white powder. All supernatants were combined and dried under nitrogen for analysis of LLO and FOS. Protein content of the powder was determined by BCA assay (Pierce). N-linked glycans were harvested from the protein powder as previously described [53] . Generally, 2 mg of protein powder (dry weight) was resuspended and digested with trypsin/chymotrypsin. Glycopeptides were enriched by Sep-Pak C18 cartridge chromatography and subjected to digestion with PNGase F for 18 h at 37 °C. Released oligosaccharides were separated from residual peptide by Sep-Pak C18 clean-up and permethylated before mass spectrometric analysis [54] . For analysis of LLO and FOS, the dried supernatants from the cell extraction were resuspended in 50% aqueous methanol and loaded onto a Sep-Pak C18 column previously washed with methanol and equilibrated in water. FOS was collected in the run-through and a subsequent water wash, which were combined and dried. The collected FOS fraction was permethylated for analysis by MS [54] . The LLOs remained bound to the Sep-Pak C18 column and were recovered by elution with methanol and 10:10:3::chloroform:methanol:water as previously described [55] . Briefly, after drying, the LLO fraction was resuspended in 10:10:3 and applied to a DEAE-cellulose column. Following washes with 10:10:3 to remove neutral lipids, the LLOs were eluted in 10:10:3 containing 300 mM ammonium acetate. The eluted LLOs were recovered by phase partition into the organic layer, which was dried and resuspended in 0.1 M HCl in isopropanol. The LLO oligosaccharides were released from dolichol pyrophosphate by heating at 50 °C for 1 h. After cooling and drying under nitrogen, the released LLO oligosaccharides were resuspended in water and recovered in the aqueous phase after addition of n-butanol. The LLO oligosaccharides in the aqueous phase were dried by lyophilization and permethylated for analysis by MS [54] . Permethylated N-linked, FOS and LLO glycans were analysed by nanospray ionization mass spectrometry using an ion trap instrument (NSI-LTQ Orbi Discoverer, Thermo-Fisher) by dissolving in 1 mM NaOH in 50% methanol and directly infusing into the instrument at a syringe flow rate of 0.40–0.60 μl min −1 . For fragmentation by CID in MS/MS and MS n modes 40% collision energy was applied. The total ion mapping functionality of the XCalibur software package (version 2.0) was utilized to detect and quantify the prevalence of individual glycans in the total glycan profile. Most permethylated oligosaccharides were identified as singly, doubly and triply charged species by NSI-MS. Total ion mapping peaks for all charge states of a given ion with m/z ≤2000 were summed together for quantification. Glycan quantification was performed relative to a known quantity of external standards (maltotriose and maltotetraose, Supelco) that was permethylated with heavy methyliodide ( 13 CH 3 I) and spiked into the sample matrix. Pulse-chase labelling and immunoprecipitation HeLa cells growing in 60 mm dishes were incubated in methionine/cysteine-free DMEM (Invitrogen) for 1 h and labelled with 1 ml of medium containing 250 μCi ml −1 TRANS 35 S-LABEL [ 35 S] (MP BIOMEDICALS) for 1 h. After washing with PBS, the cells were collected either immediately on ice or after incubation in 4 ml complete growth medium containing 2 mM L -cysteine and L -methionine for the indicated time periods. To lyse the cells, 0.8 ml lysis buffer (PBS containing 1 mM CaCl 2 , 0.5 mM MgCl 2 , 1% TritonX-100, protease inhibitor cocktail and 1 μM pepstatin A) was added. After centrifugation at 14,000 r.p.m. for 15 min, the protein concentration of the supernatant was measured using a Bio-Rad protein assay (Bio-Rad Laboratories, CA). The cell lysates (2 mg) were immunoprecipitated with 50 ng of the α5 integrin antibody BIIG2 and 60 ng of the β1 integrin antibody P5D2 overnight at 4 °C. The antibodies were precipitated with 30 μl protein G beads (Roche Diagnostics GmbH, Germany) at 4 °C for 2 h. The beads were washed five times with lysis buffer, and the immunoisolated materials were eluted by boiling for 5 min in non-reducing SDS sample buffer. Integrins were resolved using 6.5% non-reducing SDS–polyacrylamide gel electrophoresis. To determine whether the marker proteins interact with GRASP55 or GRASP65, HeLa cells or HeLa cells infected with VSV-G ts045-GFP adenovirus for 20 h, were lysed in 20 mM Tris-HCl, pH7.4, 150 mM NaCl, 1% Triton X-100, 25 mM β-glycerolphosphate and protease inhibitors. Lysate was cleared by centrifugation and mixed with antibodies to β1 integrin, Lamp1, Lamp2, GM130 or GFP and subsequently isolated by protein A or protein G beads followed by western blot analysis. Annexin V assay HeLa cells grown on cover slides were incubated with annexin V-EGFP diluted 1:100 in the binding buffer provided by the manufacturer (BioVision, K104-25) at room temperature in the dark. After washing with PBS, the cells were fixed, permeabilized and stained with Hoechst 33342. Images were taken using a Zeiss Observer Z1 inverted microscope with a × 40 lens. Quantification and statistics In all figures, the quantification results are expressed as the mean±s.e.m. (s.e. of the mean) from three independent experiments, unless otherwise stated. The statistical significance of the results was assessed using a Student’s t -test. * P< 0.05, ** P <0.01, *** P <0.001. For glycomic analysis, individual biological samples were analysed twice, once without external standard and once following addition of standard. The five most abundant high-mannose glycans and the three most abundant complex glycans were quantified relative to the external standard. Fold changes relative to normal cells were calculated for each glycan and statistical differences between the fold changes for the group of high-mannose and complex glycans were determined using a Student’s t -test, ** P <0.01. How to cite this article: Xiang, Y. et al . Regulation of protein glycosylation and sorting by the Golgi matrix proteins GRASP55/65. Nat. Commun. 4:1659 doi: 10.1038/ncomms2669 (2013).